Analysis of elite variety tag SNPs reveals an important allele in upland rice Elite crop varieties usually fix alleles that occur at low frequencies within non-elite gene pools. Dissecting these alleles for desirable agronomic traits can be accomplished by comparing the genomes of elite varieties with those from non-elite populations. Here we deep-sequence six elite rice varieties and use two large control panels to identify elite variety tag single-nucleotide polymorphism alleles (ETASs). Guided by this preliminary analysis, we comprehensively characterize one protein-altering ETAS in the 9- cis -epoxycarotenoid dioxygenase gene of the IRAT104 upland rice variety. This allele displays a drastic frequency difference between upland and irrigated rice, and a selective sweep is observed around this allele. Functional analysis indicates that in upland rice, this allele is associated with significantly higher abscisic acid levels and denser lateral roots, suggesting its association with upland rice suitability. This report provides a potential strategy to mine rare, agronomically important alleles. Crop breeding first began with the domestication of wild plants and continued with the improvement of both landraces and elite varieties. In this context, crop breeding is essentially human-directed evolution [1] . Genetic variations within natural and breeding populations provide the raw materials for this evolution, while artificial selection of particular traits serves as the driving force [2] . The selective advantage of rare and valuable mutant genes is the key to crop domestication [1] and improvement [3] , [4] . Because agronomically important genes are unnecessary for wild strains and are usually dispensable for the non-elite landraces, they usually exist at low frequencies in non-elite populations. For example, the famous ‘green revolution genes’ Rht1 and sd1, both originally came from an extremely limited set of lines that included Norin-10 (ref. 3 ) in wheat and Dee-goo-woo-gen in rice [4] , [5] . Consequently, desired alleles are likely present only at low frequencies within the non-elite gene pool [6] , [7] . Accordingly, breeders interested in infiltrating rare alleles into targeted varieties must harness hybridization and selection—a process known as gene pyramiding [6] , [8] . Asian cultivated rice ( Oryza sativa ) was among the first domesticated cereals. Asian cultivated rice consists of two main types, O. sativa type japonica (Japonica) and O. sativa type indica (Indica), with two wild progenitors, O. rufipogon and O. nivara [9] . The domestication and subsequent localization of these crops produced many rice landraces that constitute the bulk of genetic resources for rice breeding. For different objectives, such as high yield, product quality, resistance to abiotic and biotic stresses and agronomic suitability, breeders have managed to breed numerous elite varieties carrying suitable allelic combinations. Traditionally, the identification of agronomically related genes has been conducted using quantitative trait locus (QTL)/gene mapping. This approach has facilitated great progress in identifying important genes in rice, such as Gn1a , which controls grain number [10] ; Ghd7 , which affects grain number, plant height and heading date [11] ; GS3 , which controls grain weight and length [12] ; GW5 , which influences grain weight [13] ; and DEP1 , which influences density and erectness of panicles [14] . Despite its merits, QTL/gene mapping is labour intensive and time consuming, taking years to construct segregating populations and requiring extensive phenotyping and genotyping. Conversely, another popular method, association mapping, often misses the excellent alleles, as they intrinsically tend to be rare and are difficult to detect with typical association analyses [15] , [16] . In recent years, population genomics approaches involving whole-genome scans for selective sweep regions or single-nucleotide polymorphisms (SNPs) with large frequency imbalances between populations has also been used to identify selected genes [17] , [18] , [19] , [20] , but these population genomics approaches tend to identify the common alleles and miss those elite ones selected in one or a limited number of elite varieties. In this study, we first attempt a new approach to assist in the allele mining of elite rice varieties. Our approach is predicated on using a large amount of genomics data to identify elite variety tag SNP alleles (ETASs). We then comprehensively characterize an ETAS that confers a higher abscisic acid (ABA) level and denser lateral roots, which has important functional significance in the suitability of upland rice. This study provides a new potential strategy to identify rare, agronomically important alleles. Identification of ETASs for six elite rice varieties Six elite varieties (Guichao2, Minghui63, IR64, IRAT104, Koshihikari and Chujing27) were chosen based on their agronomic importance, for example, high yield, wide regional adaptability, strong drought resistance and excellent eating and cooking quality, and each were sequenced for 15 × coverage (Methods). Published genomic data sets of two non-elite populations were used as control panels. Control panel I included 40 cultivars (mainly landraces) and 25 wild accessions [17] ( Supplementary Table S1 ), and control panel II consisted of 517 Chinese landraces [18] . We defined ETASs as SNP alleles that are fixed in an elite variety but are present at frequencies lower than 5% in both control populations. One exception is that because some accessions in control panel II were upland rice, we set the frequency threshold for upland rice IRAT104 in control panel II at 10% instead of 5% to avoid missing upland rice ETASs. To ensure the ETAS alleles we identified were fixed in a particular elite variety, we selected five individuals of different sources ( Supplementary Table S2 ) for each elite variety to eliminate within-variety polymorphism. The genomes of each individual of the six varieties were sequenced using an Illumina GA2. In total, we obtained 1.23 billion paired-end reads that passed the quality filters of the Illumina GA pipeline v1.0, amounting to 54.1G base pairs. Using short oligonucleotide analysis package (SOAP) [21] and the reference Nipponbare genome (IRGSP/RAP build 5), 1.04 billion (84.76%) reads were aligned to the Nipponbare reference sequence. For each variety, the reads covered more than 90% (ranging from 90.5 to 96%) of the reference genome. As for the genomic data of the accessions in the two control panels, each was mapped onto the Nipponbare reference genome with the same pipeline. SOAPsnp1.02 was then used to process the SOAP output, enabling us to determine the genotypes of the nucleotides along the chromosomes for each elite variety and the accessions in the control panels (see Methods). As a result, we obtained the genotype of each nucleotide site for the elite varieties and the two control populations in reference to the Nipponbare coordinates. We conducted a series of site filters to ensure that the genotype calling would be of high quality and that the control panels would be representative of the rice gene pool (Methods). Next, the allele frequency of each site in the two control panels was calculated based on the genotypes of accessions, and ETASs for each elite variety were identified (Methods). 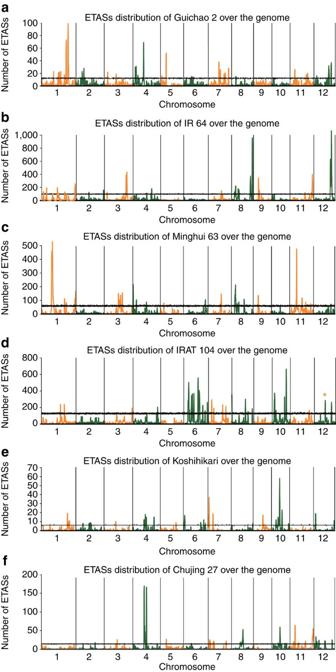Figure 1: ETAS distribution along the genomes of six elite varieties: Guichao2 (a), IR64 (b), Minghui63 (c), IRAT104 (d), Koshihikari (e) and Chujing27 (f). For each 500-kb sliding window, the number of ETASs was plotted on the entire genome. The sliding step is 50 kb. The 12 chromosomes are spaced with vertical line. Adjacent chromosomes are delineated using different colours. The horizontal black lines represent the threshold for the 95th percentile of 10,000 permutations of the ETAS numbers for all windows along the genomes. The red asterisk in the IRAT104 panel refers to the peak corresponding to theNcedlocus. In total, we identified 60,909 ETASs in the six elite varieties Guichao2 (2,598), IR64 (18,695), Minghui63 (11,411), IRAT104 (24,652), Koshihikari (914) and Chujing27 (2,639), where the parenthetical number represents the number of ETASs in each ( Table 1 ; all ETASs are presented in the Supplementary Data S1 ). Generally speaking, these ETASs appeared to be randomly distributed over the entire genome with a few enriched peaks ( Fig. 1 ). To pick out significantly ETAS-enriched regions for each variety, a permutation test was performed to derive the threshold of significance for each window (Methods). Windows with peaks higher than the local threshold are possibly enriched with targeted genes for elite rice improvement. The distribution patterns of ETASs and their enriched peaks differ from variety to variety, as they have been bred for different traits and are adapted to different growing conditions. Table 1 Summary of ETASs in the six elite varieties. Full size table Figure 1: ETAS distribution along the genomes of six elite varieties: Guichao2 ( a ), IR64 ( b ), Minghui63 ( c ), IRAT104 ( d ), Koshihikari ( e ) and Chujing27 ( f ). For each 500-kb sliding window, the number of ETASs was plotted on the entire genome. The sliding step is 50 kb. The 12 chromosomes are spaced with vertical line. Adjacent chromosomes are delineated using different colours. The horizontal black lines represent the threshold for the 95th percentile of 10,000 permutations of the ETAS numbers for all windows along the genomes. The red asterisk in the IRAT104 panel refers to the peak corresponding to the Nced locus. Full size image Identifying protein-altering ETASs SNP mutations causing protein-coding changes or gene expression alterations both have the potential to account for agronomic traits [22] . In addition, unlike during domestication, in crop improvement, a larger proportion of mutations involved are protein altering rather than regulatory changes [22] , [23] . Furthermore, considering the difficulty in defining whether an ETAS alters expression, to narrow down the ETASs to those with biological importance, we mainly focused on protein-altering ETASs. We used genomic annotation to assign sites to different categories related to transcription and translation, including genic regions (coding DNA sequences (CDSs), introns and untranslated regions (UTRs)), promoter regions (the upstream 300 bp before a transcription start site) and intergenic regions ( Table 1 ). We defined ‘protein-altering’ ETASs as those that result in premature stop codons, disrupt start/stop codons or splice donor/acceptor sites, or are non-synonymous mutations ( Table 1 ). These mutations have the potential to generate strong functional effects associated with the elite agronomic traits of a particular plant variety. The protein-altering ETAS in the Nced gene of upland rice Among the protein-altering ETASs, those occurring in the upland rice IRAT104 were further analysed because the hallmark of this variety, drought resistance, is especially significant to impoverished upland communities. Interestingly, among the several hundred protein-altering ETASs, we noted a non-synonymous mutation at site 14390318 (C->T) on chromosome 12 of upland rice IRAT104 located within the 9- cis -epoxycarotenoid dioxygenase gene ( Nced, Os12g0435200 ). This previously unreported mutation results in an amino-acid change from valine to isoleucine. Nced encodes a rate-limiting key enzyme in the ABA biosynthetic pathway [24] and has been reported to be associated with dehydration tolerance in Arabidopsis [25] and beans [26] . We examined the occurrence of the T-type allele in the control panels and found that all 61 accessions in control panel I with sequence reads at this locus bear the C-type allele, and 38 accessions in control panel II have the T-type allele. We were surprised to find that 37 of the 38 T-type accessions in the control panel II were upland rice ( Supplementary Table S3 ). To test the association of this SNP with upland rice, we expanded our sample size to include 109 upland and 102 irrigated rice varieties ( Supplementary Table S4 ) and genotyped this SNP using a cleaved amplified polymorphic sequence marker [27] . This genotyping experiment resulted in an allele frequency for the T-type allele of 61% in upland rice but a frequency of only 3% in irrigated rice ( Supplementary Fig. S1 , Supplementary Table S4 ). The dramatic allele frequency difference between upland and irrigated rice strongly indicates that the T-type allele may be associated with adaptation to the upland environment and that human-guided artificial selection during upland rice breeding has likely increased its frequency. Because the varieties we chose occur over a wide geographic distribution (indicated by the blue dots in Supplementary Fig. S2 ) and both the upland and irrigated groups consist of strains belonging to Indica and Japonica types ( Supplementary Table S4 ), it is less likely that population structure would undermine the association between the Nced ETAS and upland rice. To further test whether Nced has indeed undergone selection within upland rice varieties, we calculated the average nucleotide diversity levels ( π (ref. 28 )) of this gene and its 2-Mb flanking regions on both sides using our genome resequencing data of 84 upland and 82 irrigated rice varieties ( Supplementary Table S4 ). We divided the upland rice population into group I with the C-type allele and group II with the T-type allele to determine whether a selective sweep occurred for the T-type allele in upland rice. As illustrated in Fig. 2a , the T-type upland group has obviously low diversity around the Nced gene, whereas the C-type upland and irrigated rice cultivars have relatively normal diversity levels compared with the adjacent genomic regions. This apparent sweep resulted in a ~350-kb linkage disequilibrium region in the T-type upland rice ( Fig. 2a ). 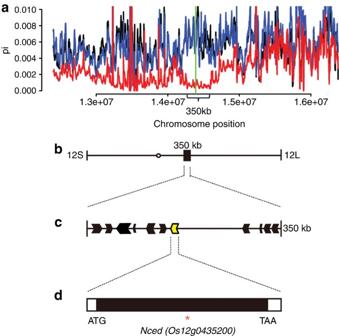Figure 2: Illustration of the 350-kb selective sweep region. Nucleotide diversity (π) is the number of nucleotide differences per site between two randomly chosen sequences of upland and irrigated rice (see Methods). (a) Selective sweep signals around theNcedgene. The horizontal axis shows the coordinates on chromosome 12. For example, ‘1.4e+07’ refers to the coordinate ‘14,000,000’. The vertical axis indicatesπvalues. The red, blue and black curves indicateπvalues of the T-type upland population, C-type upland population and irrigated population, respectively. The green vertical line marks the position of theNcedgene. (b) A 350-kb selective sweep region on chromosome 12; ‘12S’ and ‘12L’ indicate the short and long arms of chromosome 12, respectively. (c) Eleven genes in the 350-kb region; the yellow arrow is theNcedgene. (d) The protein-altering ETAS inNcedis indicated with a red asterisk. Figure 2: Illustration of the 350-kb selective sweep region. Nucleotide diversity ( π ) is the number of nucleotide differences per site between two randomly chosen sequences of upland and irrigated rice (see Methods). ( a ) Selective sweep signals around the Nced gene. The horizontal axis shows the coordinates on chromosome 12. For example, ‘1.4e+07’ refers to the coordinate ‘14,000,000’. The vertical axis indicates π values. The red, blue and black curves indicate π values of the T-type upland population, C-type upland population and irrigated population, respectively. The green vertical line marks the position of the Nced gene. ( b ) A 350-kb selective sweep region on chromosome 12; ‘12S’ and ‘12L’ indicate the short and long arms of chromosome 12, respectively. ( c ) Eleven genes in the 350-kb region; the yellow arrow is the Nced gene. ( d ) The protein-altering ETAS in Nced is indicated with a red asterisk. Full size image Demographic events, such as breeding bottlenecks, could have resulted in the low diversity around the T-type Nced locus. Using sequence data from the upland and irrigated populations for the ~350-kb region and its right flanking sequence, we constructed phylogenetic trees for these accessions ( Supplementary Fig. S3 ). The results indicate that in the ~350-kb region, the T-type upland accessions form a monophyletic group, whereas for the flanking sequence, the T-type upland accessions mix with the C-type upland and irrigated accessions. Because demographic effects usually influence the entire genome, if the low-diversity region around the T-type Nced allele were due to demographic effects, the tree for this region would display a similar pattern with the tree for its flanking sequence. The above analyses demonstrate that diversity recovers rapidly outside the ~350-kb low-diversity region, suggesting that artificial selection is more likely than demography to have caused the low diversity around the Nced gene. Genes within the 350-kb selective sweep region There are only 11 genes within the 350-kb low-diversity region ( Fig. 2c , Table 2 ), with the Nced gene located near the centre ( Fig. 2c ). In this region of IRAT104, there are a total of 263 ETASs, of which only two are protein altering ( Table 2 ). One of the protein-altering ETASs is in the Nced gene; the other is located in the gene Os12g0435000 , resulting in a nonsense mutation in some upland accessions with 27 amino acids truncated from the C terminus of the predicted protein. The frequency difference between upland and irrigated rice for this ETAS is only 23%, much less than the 58% difference for the non-synonymous ETAS in the Nced gene. Likewise, functional annotation of Os12g0435000 indicates that it encodes a zinc finger protein, but there is no supporting evidence that this function is related to upland adaptability. Moreover, although there is no available mutant for the Nced gene, we did obtain one homozygous T-DNA insertion mutant for the neighbouring gene Os12g0435000 from the TRIM library of Taiwan. However, no visible phenotypic difference in upland environment was observed for this mutant when we compared it with the wild type ( Supplementary Fig. S4 ). For these reasons, it appears that the ETAS truncating the Os12g0435000 gene, along with those non-protein-altering ETASs, may have hitch-hiked with the protein-altering ETAS in the Nced gene from the selective sweep for the T-type Nced allele. Table 2 Eleven genes in the 350-kb selective sweep region around the Nced . Full size table We also checked the expression patterns of the Nced and Os12g0435000 genes using semi-quantitative PCR of three tissues (stem, leaf and root) across nine varieties (Methods). The Nced gene was expressed in all of these tissues in these varieties, whereas the expression level of Os12g0435000 was almost undetectable ( Supplementary Fig. S5 ). We then surveyed the spatial-temporal expression pattern of the Nced gene using quantitative PCR. The Nced gene was expressed mainly in leaves during the vegetative stage after tillering, although stems in the vegetative stage after tillering and roots in the reproductive stage similarly displayed moderate expression ( Supplementary Fig. S6 ). The Nced ETAS is associated with an ABA increase Functional data provides better evidence to support or reject the hypothesis that selection for the Nced allele occurred. Because the Nced gene encodes the key enzyme for catalysing ABA synthesis, we speculated that the T-type allele in upland rice might have altered the catalytic efficiency of this enzyme, resulting in an altered level of ABA synthesis. Through in silico prediction, we found that the amino-acid substitution changed the protein’s secondary structure around the nearby binding sites ( Supplementary Fig. S7 ), strongly suggesting it might have altered the enzyme activity. To further test this speculation, we chose 20 T-type upland rice varieties and 17 C-type upland varieties to measure their ABA levels in leaves during the vegetative stage after tillering by enzyme-linked immunosorbent assay (ELISA) ( Supplementary Table S5 ). Interestingly, the results indicate that the ABA levels of T-type upland rice are significantly higher than those of C-type upland rice ( t -test, P =0.033, Fig. 3a ). Furthermore, we managed to obtain an F7 segregating population of recombinant inbred lines (RILs) constructed by crossing IR64 (C-type) and IRAT104 (T-type). This RIL population has 23 families (12 C-type and 11 T-type). We measured the ABA levels of the C-type and T-type families ( Supplementary Table S6 ) and found that T-type families have consistently higher ABA levels than C-type ones ( t -test, P =0.016, Fig. 3b ). As a well-known stress hormone, ABA has been frequently reported to enhance drought resistance in plants [25] , [26] . Thus, our observations suggest that the T-type allele of the Nced gene likely confers greater drought resistance on upland rice by raising endogenous ABA levels. Plants have various drought resistance mechanisms: drought escape, dehydration avoidance and dehydration tolerance [29] , [30] . ABA can be involved in both constitutive dehydration avoidance and inducible dehydration tolerance [31] . There is evidence that drought resistance mechanisms in upland rice depend more on constitutive dehydration avoidance through water absorption by a developed root system than on inducible dehydration tolerance, such as osmotic adjustment responses to maintain water potential [32] , [33] , [34] . Accordingly, we wondered whether the ABA-increasing ETAS also enhances the root system, further improving performance in dry conditions. 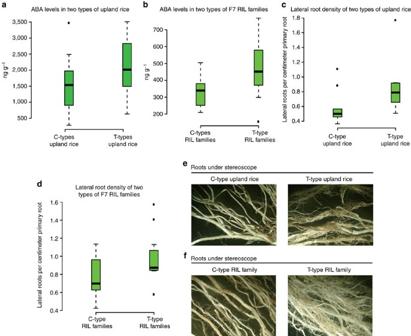Figure 3: Association ofNcedalleles with ABA levels and lateral roots. (a) Box plot of ABA levels of 17 C-type and 20 T-type upland varieties. The vertical axis indicates the ABA contents. The ABA level of T-type upland rice is significantly higher than that of C-type upland rice (t-test,P=0.033). (b) The ABA levels of 12 C-type and 11 T-type families in the F7 RIL population. T-type families have significantly higher ABA levels (t-test,P=0.016). (c) Comparison of the lateral root densities of 9 C-type and 8 T-type upland varieties showing that T-type upland varieties have denser lateral roots than C-type varieties (t-test,P=0.009). (d) Comparison of the lateral root densities between the 12 C-type and 11 T-type families in the RIL population showing that T-type families have denser lateral roots (t-test,P=0.035). (e,f) Root system observations under stereoscope of the C-type upland variety IRAT 12 and the T-type upland variety Honghangu, and the C-type family DT51 and T-type family DT81 from the RIL, respectively. For box plots, the bottom, top and middle bands of the boxes indicate the 25th, 75th and 50th percentiles, respectively. Whiskers extend to the most extreme data points no more than 1 interquartile in range from the box. The empty circles are the extreme values. Figure 3: Association of Nced alleles with ABA levels and lateral roots. ( a ) Box plot of ABA levels of 17 C-type and 20 T-type upland varieties. The vertical axis indicates the ABA contents. The ABA level of T-type upland rice is significantly higher than that of C-type upland rice ( t -test, P =0.033). ( b ) The ABA levels of 12 C-type and 11 T-type families in the F7 RIL population. T-type families have significantly higher ABA levels ( t -test, P =0.016). ( c ) Comparison of the lateral root densities of 9 C-type and 8 T-type upland varieties showing that T-type upland varieties have denser lateral roots than C-type varieties ( t -test, P =0.009). ( d ) Comparison of the lateral root densities between the 12 C-type and 11 T-type families in the RIL population showing that T-type families have denser lateral roots ( t -test, P =0.035). ( e , f ) Root system observations under stereoscope of the C-type upland variety IRAT 12 and the T-type upland variety Honghangu, and the C-type family DT51 and T-type family DT81 from the RIL, respectively. For box plots, the bottom, top and middle bands of the boxes indicate the 25th, 75th and 50th percentiles, respectively. Whiskers extend to the most extreme data points no more than 1 interquartile in range from the box. The empty circles are the extreme values. Full size image Denser lateral roots associate with the ABA-increasing ETAS Our pilot phenotypic survey in several accessions suggested that lateral roots differ between C-type and T-type upland rice. To confirm these findings, we conducted two experiments designed to test the association between the ETAS and lateral root system. First, we grew 9 C-type upland varieties and 8 T-type upland varieties (five individuals for each variety). When they were in the vegetative stage after tillering, we investigated their phenotypes (Methods) and noted that the average number of lateral roots per centimetre main root of T-type upland rice was significantly larger than that of C-type upland rice ( t -test, P =0.009) ( Fig. 3c and Supplementary Table S7 ). We also phenotyped the lateral root density in the F7 RIL population constructed by crossing IRAT104 and IR64. T-type families also display significantly denser lateral roots than C-type families ( t -test, P =0.035) ( Fig. 3d and Supplementary Table S8 ). These data suggest that the T-type Nced allele might have had a crucial role in generating this adaptive phenotype in T-type upland rice by elevating ABA levels. Comparing ETAS analysis with population genomics analysis To test whether ETAS analysis has some unique advantages in guiding rare allele mining, we also used a population genomics approach to identify possible selected genes in upland rice using whole-genome resequencing data of 84 upland and 82 irrigated rice varieties. After SNP calling, we calculated the allele frequencies of each SNP for the two populations (Methods). A previous work used a threshold of allele frequency difference of 0.8 to screen the selected regions [19] . In our study, when using the threshold of 0.8, we obtained 6,369 frequency-differentiated SNPs without the Nced ETAS, which we observed has an allele frequency difference of 0.58 between the upland and irrigated population. Even when a less stringent threshold (0.5) was used, among the long list of 90,076 SNPs, the Nced ETAS has a very low ranking. We then further conducted a whole-genome scan for selective sweep regions that were determined by taking those windows with the highest 5% of values for reduction of diversity [17] (ROD, Methods) of the upland population compared with the irrigated population, yielding a list of 1,362 genes ( Supplementary Data S2 ), again among which the Nced gene was not found. While in general, these frequency-differentiated SNPs and potentially selected genes might be useful in identifying genes important to rice upland adaptation and evolution, these results indicate that our ETAS approach can be a useful guide in identifying elite alleles. In this study, we identified ETASs to guide allele mining in elite varieties. The observation that Japonica varieties tend to have fewer ETASs than Indica varieties is most likely because there is much less population variation in Japonica compared with Indica [9] . The odd result that indica Guichao2 has far fewer ETASs is perhaps due to the sequence coverage bias of this variety. When we used a depth of 5 as the filtering cutoff (Methods), we removed the majority of ETASs in this variety ( Supplementary Table S9 ). The only upland rice of the six varieties, IRAT104, possesses the most ETASs, most likely because of its special upland ecotype resulting from its distinctive breeding process and the looser threshold used to identify ETASs in this variety. These facts indicate that breeding histories may have a great effect on the ETAS numbers of elite varieties. Along with breeding histories, control panels also have an effect on ETAS numbers. Some of the ETASs may not turn out to be rare and can be excluded as the control panels expand, but ETASs actually associated with elite characteristics that are rare in the control panels should be retained. Moreover, it is worth noting that some varieties with the same agronomic trait may share the same ETASs, just like the ETAS in the Nced gene, which is shared by most upland rice varieties. Many previously identified alleles associated with advantageous agronomic traits turned out to be SNPs causing amino-acid changes, premature stop codons and disruptions of start/stop codons or splice donor/acceptor sites. For example, ehd1 and hd6 , which affect flowering time, result from a Gly-to-Arg amino-acid change [35] and a premature stop codon [36] , respectively. The Japonica semi-dwarf gene, sd1, results from an amino-acid substitution at the conserved residue Leu-266 (ref. 37 ), and its counterpart, Rht1 , in semi-dwarf wheat, is the result of a premature stop codon [38] . Moreover, waxy, which causes sticky grains, results from an intron-splicing defect [39] . These empirical studies have shown that protein-altering SNPs might be associated with agronomic traits. In our study, we identified a few such protein-altering ETASs for the six elite varieties, providing a valuable checklist for screening potentially targeted genes during elite rice improvement. In screening the protein-altering ETASs of the upland rice IRAT104, we observed a dramatic frequency difference in the protein-altering ETAS in the Nced gene between upland and irrigated populations (61% versus 3%) and a low-diversity haplotype block around the ETAS. Population genomics and phylogenetic analyses indicate that the pattern is most likely the result of a selective sweep resulting from artificial selection rather than a bottleneck effect. Functional analysis of the Nced protein-altering ETAS demonstrated that it is associated with considerably increased ABA in T-type rice compared with C-type rice. Previously, ABA’s role in root growth has been controversial because ABA signalling can act as both a positive and a negative factor in root development [31] , [40] . Studies with an ABA-deficient mutant with a growth retardation phenotype of lateral roots and an ABA-insensitive mutant with a defect of lateral root initiation indicate that endogenous ABA has an essential part in promoting lateral root formation [31] , [41] , [42] . However, it has also been reported that exogenous application of ABA to wild-type plants inhibits lateral root formation [43] . From these data, we can only speculate that ABA’s function in root development most likely depends on both dose and circumstances, and most case studies indicate that endogenous ABA signalling is critical for lateral root growth. Knowing that T-type upland rice plants display higher levels of endogenous ABA synthesis, we wanted to determine whether they possess a root system with more lateral roots than present in C-type upland rice plants. We were able to demonstrate that higher endogenous ABA levels in T-type upland varieties and T-type RIL families corresponds to more lateral roots than in their C-type counterparts, suggesting that the T-type allele promotes upland rice root branching. However, it cannot be ruled out that, to some degree, the higher ABA-synthesis machinery in T-type upland rice may also result in better osmotic adjustment and stomatal regulation. Higher ABA levels can promote stomatal closure and enhance the water use efficiency of plants [44] , [45] . Thus, the T-type allele may confer higher water use efficiency in upland rice. Moreover, one known effect of ABA is that it can modulate aquaporin expression and activity, and in doing so, enhance the total hydraulic conductivity between the soil and the plant, promoting leaf rehydration and recovery of elongation [17] . Hence, an Nced enzyme with higher activity may also lead to the swifter regulation of aquaporin activity and maintenance of favourable plant water potential. In this study, we also conducted a whole-genome scan for SNPs with large allele frequency differences between upland and irrigated populations and selective sweep regions in the upland population. The fact that the yielded candidate lists did not include the Nced gene illustrates how this traditional population genomics approach tends to identify those alleles that have been fixed or are close to being fixed in a given population. These alleles are undoubtedly interesting for investigating the general evolution and adaptation of upland rice, but alleles with moderate frequency differences between populations may be missed by traditional population genomics approaches. For this reason, though ETAS preliminary analysis provides a list of candidates that need further validation, the elite agronomical alleles it may potentially discover makes it a viable technique to use, especially when the purpose is identifying rare elite alleles. In conclusion, using whole-genome deep resequencing of six elite varieties and comparing these data with large quantities of control population genomics data, we were able to identify many ETASs that are rare in most control cultivars and wild rice varieties. Our deep analyses of one protein-altering ETAS in the distinguished upland rice variety IRAT104 indicates that humans may have strongly selected this ETAS to enhance the suitability of upland rice by raising the ABA level and, in doing so, promoting lateral root density. These results suggest that the ETAS-guiding allele mining approach can be useful in identifying agronomically important genes in elite crop varieties. With the rapid advent of sequencing technology and the accumulation of extensive genomic data for more crops, we expect this approach to have a broad utility in identifying agronomically important genes in improved rice and other crops. Sample collection and DNA preparation In this study, we selected six elite varieties on the basis of their agronomic importance. Guichao2 is an indica with an extraordinarily high yield. Minghui63 is the most widely used indica male sterile restorer in China and is well known for its excellent restoration capacity and resistance to rice blast. IR64, developed by the International Rice Research Institute, is one of the most widely cultivated varieties of indica in the world and is known for its wide adaptability and high yield [46] . IRAT104, developed by the Research Institute for Tropical Agriculture and Food Crops (IRAT), is a famous upland rice variety of japonica possessing good yield under drought [47] . Koshihikari, a renowned japonica variety developed by Japanese breeders, has an exceptional aromatic and unparalleled sweet flavour. The last variety we examined, Chujing27, released by the Yunnan Province of China, is a cultivar of japonica known for its high yield and wide adaptability. For each elite variety, five individuals were collected from different sources ( Supplementary Table S2 ). We also used 84 upland and 82 irrigated rice varieties to conduct population genetics analysis ( Supplementary Table S4 ). Genomic DNA was extracted from the leaves of the trefoil-stage seedlings using a Qiagen DNeasy Plant Mini Kit. Reads mapping After high-throughput sequencing using an Illumina Genetic Analyser and removing sequencing adaptors, we obtained 1.23 billion raw reads that passed the quality filters of the Illumina GA pipeline v1.0. The raw reads of the major control panel I came from our previous work (NCBI Short Read Archive accession code SRA023116 ) (ref. 17 ). The reads of control panel II were downloaded from the NCBI SRA database (accession code ERP000106 ) (ref. 18 ). The IRGSP 5.0 Nipponbare genome was downloaded from the RAP-DB database ( http://rapdb.dna.affrc.go.jp/download/latest/IRGSPb5.fa.masked.gz ) and was used as the reference genome. Using SOAP2.20 (ref. 21 ), we mapped the raw reads to the reference genome. Because different elite varieties can have completely different elite SNP alleles, we mapped each variety separately. For each elite variety, we pooled reads of the five individuals together when mapping. We also mapped the short reads of each accession of control panels, upland and irrigated populations onto the Nipponbare genome with the same pipeline. Counting base frequencies The genotype of each nucleotide in each variety or accession was determined using SOAPsnp1.02 (ref. 48 ) ( Supplementary Methods ). To make the control group more representative for the rice gene pool, only the nucleotide sites sequenced in more than 30 accessions in both of the two control panels were retained. Moreover, because control panel I consisted of 15 Oryza rufipogon , 10 Oryza nivara , 10 indica, 10 tropical japonica, 8 temperate japonica, 4 aus, 5 aromatic and another 3 accessions with admixed backgrounds ( Supplementary Table S1 ), we eliminated the sites at which the numbers of sequenced accessions in each subpopulation deviated significantly from the random sampling expectation (chi-squared goodness-of-fit test, α <0.05) to ensure the representativeness of sampling. The base frequencies of the two control panels at each site were calculated based on the genotype of each accession. Identifying high-quality ETASs and ETAS-enriched peaks SOAPsnp1.02 provided the genotype information for each nucleotide and its sequencing depth. Considering that heterozygous sites are less likely to account for the unique and stable characteristics of a single inbred elite variety, we filtered out all heterozygous sites within each elite variety using an in-house Perl script. To make the ETASs accurate, only the sites with depths ≥5 were retained and used for further analyses. We then conducted whole-genome scans by recording the fixed genotype at a single site of an elite variety and checking its frequencies in both control panels. A SNP allele was defined as an ETAS if it was fixed in one elite variety but with frequencies <5% in both control panels. Because some accessions in control panel II were upland rice, we set the frequency threshold in the control panel II for IRAT104 at 10% instead of 5% so that we could identify more ETASs related to upland rice adaptability. To identify the ETAS-enriched windows, we performed a permutation test to obtain the significance threshold by randomly shuffling the ETAS numbers of all 500-kb sliding windows along the entire genome 10,000 times using our in-house Perl script. We set the 95th percentile of ETAS numbers of permutation tests in each window as the local threshold value (indicated by a black horizontal threshold line in Fig. 1 ). Genomic and phylogenetic analysis for Nced nearby regions A targeted gene that humans have favourably selected to enhance agricultural characteristics usually has a low level of variation and a skewed allele frequency spectrum compared with unlinked unselected regions. We resequenced the entire genomes of 82 irrigated accessions and 84 upland accessions (including 29 C-type upland accessions, 41 T-type upland rice accessions and 13 upland accessions with no reads at the Nced ETAS) using an Illumina GA2 (the resequencing data were deposited in the NCBI Short Read Archive with accession code SRA066116 ). The reads of each 2-Mb flanking region around the Nced gene were extracted for all of these accessions using in-house Perl scripts on the basis of mapping results from the SOAP software and were used to calculate the numbers of nucleotide differences per site between two randomly chosen sequences (nucleotide diversity levels, π ) (ref. 28 ) in this region. Sliding 20-kb windows were used during the calculation with a 2-kb sliding step. By comparing the diversity levels around the Nced gene among the irrigated, C-type upland and T-type upland rice groups, we were able to see the signature of selection in the T-type upland rice ( Fig. 2 ). The reads within the 350-kb low-diversity region and its right flanking region were used to calculate the pairwise distances for the accessions, respectively, and then construct the neighbour joining trees using PHYLIP (ref. 49 ). Origin of mutant and RIL materials The mutant M0002772 was bought from the TRIM library of Taiwan, and the RIL population was provided by Yunnan Academy of Agricultural Sciences. Measuring ABA levels with ELISA We chose 20 T-type upland rice varieties and 17 C-type upland varieties to measure ABA levels using an ELISA ( Supplementary Table S5 ). The plants were planted in flower pots (~10 individuals for each pot) under a simulated upland environment (controlling water to prevent submergence). Each sample consisted of ~0.5 g of fresh leaves of vegetative stage individuals after tillering. We selected leaf tissue at this stage because, according to quantitative PCR results, the Nced gene displays its highest expression level at this stage ( Supplementary Fig. S6 ). Each sample was pulverized in liquid nitrogen using a mortar and pestle and was then extracted with 80% methanol (including 1 mmol l −1 butylated hydroxytoluene, BHT) at 4 °C overnight. The mixture was centrifuged at 5,000 g for 15 min. The supernatant was blow-dried with nitrogen and dissolved in phosphate buffer (pH 7.5, 1% Tween-20, 1% glutin). The measurement of each sample’s ABA level was then conducted using an ELISA. The primary antibody, a monoclonal mouse antibody, was provided by Dr Baoming Wang’s lab of the China Agricultural University. The coupling reaction for the secondary antibody was performed using the standard horseradish peroxidase method [50] . Quantifying lateral roots We chose 9 C-type upland accessions and 8 T-type upland accessions and grew them in flower pots (five individuals for each pot) in a simulated upland environment (controlling water from submergence). When the seedlings were in the vegetative stage after tillering, we pulled them out of the soil as gently as possible without damaging the root systems and washed the roots clean to measure the lengths of all of the main adventitious roots. We then counted the lateral roots that branched from the main roots. To reduce the workload, we counted only the lateral roots longer than 1 cm. Lateral root density was calculated by dividing the total lateral root number by the total main root length. For each variety, we quantified lateral root density for five individuals and calculated the mean value. We used the same method to quantify the lateral roots of the C-type and T-type families in the RIL population. Population genetics analysis for two populations We used SOAPsnp1.02 to call SNPs for the entire populations of the irrigated and upland accessions [48] . A filtering series was conducted to ensure SNP quality. For example, SNPs with quality values <15 or with nearby copy numbers >1.5 were removed. We also eliminated SNP sites with depths less than 6 or greater than 300. SNP allele frequencies in each population were calculated based on the SNP genotypes of each accession. The nucleotide diversity level, π , was calculated using the method mentioned above. Sliding 20-kb windows were used during the calculation with a 2-kb sliding step. ROD was computed using the formula, ROD=( π irrigated −π upland )/ π irrigated . Accession codes: The raw sequence data of the 30 individuals of the six elite varieties have been deposited into the NCBI Short Read Archive (SRA, http://www.ncbi.nlm.nih.gov/sra/ ) under the accession code SRA035256 . The reads of the 84 upland and 82 irrigated rice accessions ( Supplementary Table S4 ) have been deposited into the NCBI Short Read Archive under the accession number SRA066116 . How to cite this article: Lyu, J. et al . Analysis of elite variety tag SNPs reveals an important allele in upland rice. Nat. Commun. 4:2138 doi: 10.1038/ncomms3138 (2013).